Fossil pollen records indicate that Patagonian desertification was not solely a consequence of Andean uplift The Patagonian steppe—a massive rain-shadow on the lee side of the southern Andes—is assumed to have evolved ~15–12 Myr as a consequence of the southern Andean uplift. However, fossil evidence supporting this assumption is limited. Here we quantitatively estimate climatic conditions and plant richness for the interval ~10–6 Myr based on the study and bioclimatic analysis of terrestrially derived spore–pollen assemblages preserved in well-constrained Patagonian marine deposits. Our analyses indicate a mesothermal climate, with mean temperatures of the coldest quarter between 11.4 °C and 16.9 °C (presently ~3.5 °C) and annual precipitation rarely below 661 mm (presently ~200 mm). Rarefied richness reveals a significantly more diverse flora during the late Miocene than today at the same latitude but comparable with that approximately 2,000 km further northeast at mid-latitudes on the Brazilian coast. We infer that the Patagonian desertification was not solely a consequence of the Andean uplift as previously insinuated. The Miocene Andean uplift has had a far-reaching influence on the evolution of South American landscapes and ecosystems [1] , [2] . The climatic, biodiversity and environmental response to this orographic forcing is well understood in northern South America [3] , [4] but virtually unknown in southern South America (Patagonia). The uplift of the Patagonian Andes appears to have caused an extraordinary rain-shadow on the leeward—present Patagonian steppe—since ~14–12 Myr according to tectonic and isotopic evidence [5] , [6] , [7] . However, fossil-derived data supporting this regional turnover are virtually absent, largely because Patagonian terrestrial sedimentation after the mid Miocene (~14 Myr) has been almost exclusively limited to short-lived episodes of coarse-grained terrestrial accumulation [7] , [8] , resulting in scattered and biologically barren deposits. Today the Patagonian steppe is South America’s largest and southernmost desert ecosystem ( Fig. 1 ). Climatic conditions are harsh ( Fig. 2 ), with low mean winter temperatures (Mean Temperature of the Coldest Quarter (MTCQ): ~3.5 °C), low precipitations (Annual Precipitations (APs): ~200 mm) and strong westerlies (15–22 km hour −1 ). Under these climatic conditions, an open grass-dominated steppe expands with sclerophyll shrub patches of Asteraceae (daisy family) and Fabaceae (bean family) as the most important families [9] . 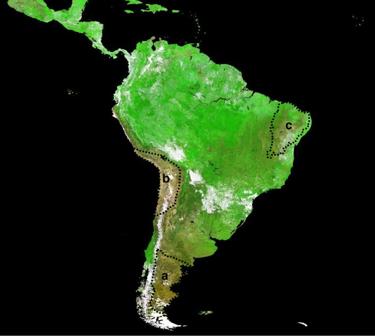Figure 1: South American vegetation map based on satellite imagery. Driest regions are indicated on the map by dashed lines: (a) Patagonian steppe, (b) Atacama desert and outlying arid areas and (c) Caatinga scrub. Map obtained by European Space Agency satellite Proba-V (June 2013). Figure 1: South American vegetation map based on satellite imagery. Driest regions are indicated on the map by dashed lines: ( a ) Patagonian steppe, ( b ) Atacama desert and outlying arid areas and ( c ) Caatinga scrub. Map obtained by European Space Agency satellite Proba-V (June 2013). 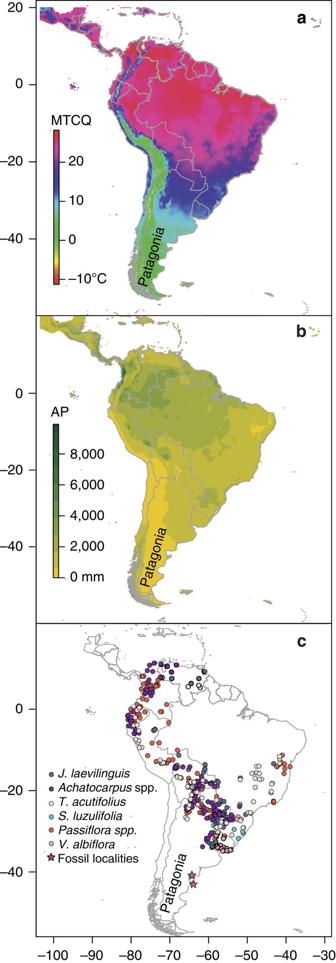Figure 2: South American maps showing bioclimatic variables and extant and fossil localities. (a,b) Maps depict two crucial bioclimatic variables for plant distribution: MTCQ (Mean Temperature of the Coldest Quarter) and AP (Annual Precipitation). (c) Map depicts the geographic distribution of fossil sites (stars) and selected nearest living relatives (circles). Note the relatively low values of MTCQ and AP in the Patagonian region. Full size image Figure 2: South American maps showing bioclimatic variables and extant and fossil localities. ( a , b ) Maps depict two crucial bioclimatic variables for plant distribution: MTCQ (Mean Temperature of the Coldest Quarter) and AP (Annual Precipitation). ( c ) Map depicts the geographic distribution of fossil sites (stars) and selected nearest living relatives (circles). Note the relatively low values of MTCQ and AP in the Patagonian region. Full size image Here we quantitatively estimate climatic conditions and plant richness (relative for sample size) for the interval ~10–6 Myr using the bioclimatic profiles of key-sensitive species and rarefaction curves from raw count data, respectively. Our estimations derived from fossil pollen grains preserved in shallow-marine sediments exposed in eastern Patagonia for which we have obtained 87 Sr/ 86 Sr ages. Our study represents a new explicit picture of late Neogene landscapes from southern South America and brings forward the timing of the onset of Patagonian desertification. Diversity patterns and palaeoclimate We identified 68 fossil pollen and spore types assigned to formally described fossil genera or species ( Supplementary Table 1 ). The actual number of plant taxa preserved is likely to be higher as many fossil types represent more than one natural species or genus. Many of the recovered fossil taxa produce relatively few pollen grains with limited dispersal capabilities (for example, most entomophilous plants), indicating that the parent plants grew close to (or upstream from) the accumulation site. The botanical affinities of fossil pollen and spore species fall into moderately distinct ecological groups that most likely grew across an estuarine gradient from lowlands (Atlantic coastal region) to highlands (Patagonian inland). These ecological groups include (1) swamp and salt-marsh communities that occupied permanently-wet soils; (2) semi-deciduous communities that occupied well-drained and/or salty soils; and (3) forest communities that occupied upstream (inland) zones. The first community includes salt-tolerant (Amaranthaceae (amaranth family), Ephedra , and Cressa (alkaliweeds)) as well as fresh and brackish water (for example, Cyperaceae (sedges), Typhaceae (bulrush), Myriophyllum (watermilfoil), Azolla (water fern), Pediastrum ) taxa. The second community includes small trees ( Achatocarpus , Prosopis , Celtis and Anacardiaceae) and probably some shrubs and herbs (for example, Chuquiraga , Nassauvia and Calyceraceae). Tropical vines, parasites and shrubs also occupied this community, probably close to watercourses (for example, Schlechtendalia , Justicia , Malpighiaceae and Loranthaceae). The third community includes wet-demanding taxa (for example, Nothofagaceae, Podocarpaceae, Winteraceae) that may have grown upstream from the accumulation site as more or less discontinuous patches on mainland Patagonia. The presence of some wet-demanding plants with very limited pollen dispersal such as Saxegothaea and Araucaria [10] supports the notion that forest prevailed upstream, towards the Patagonian interior. Rarefied curves indicate that diversity values fluctuated between 25 and 28 species per sample in 185 counted pollen grains during the interval 10–6 Myr. We compared these diversity values with those from present and older Patagonian samples ( Fig. 3a ), from coeval Amazonian samples ( Fig. 3b ) and from present SE Brazilian samples ( Fig. 3c ). We found significant differences in the overall number of species ( post hoc Tukey test, P <0.001) among all assemblages compared (in 185 counted specimens), except for those between the late Miocene of Patagonia (this study) and recent pollen-rain from SE Brazil ( post hoc Tukey test, P =0.976, Fig. 4 ). Rarefaction analysis with different sampling effort shows that there is no significant variation in within-sample diversity among the compared assemblages, regardless of sample counting intensity ( Supplementary Fig. 1 ). 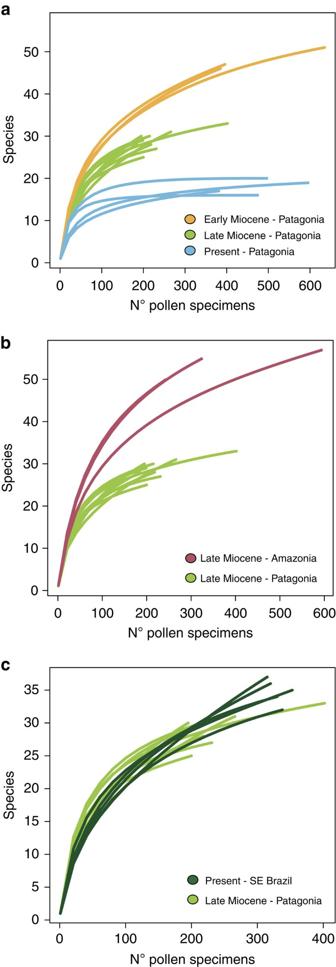Figure 3: Rarefied within sample richness based on selected fossil and extant pollen data. Curves indicate the number of expected taxa for a certain sample size (that is, number of pollen grains counted). (a) Curves contrasting the late Miocene (light-green curves) with present (light-blue curves) and early Miocene (orange curves) pollen assemblages from Patagonia. (b) Curves contrasting Patagonian (light-green curves) and Amazonian (magenta curves) pollen assemblages from the late Miocene. (c) Curves contrasting the Patagonian late Miocene (light-green curves) with SE Brazilian present (dark-green curves) pollen assemblages. For readability purposes, only the most diverse samples are shown. Note that the Patagonian late Miocene and SE Brazilian recent samples appear to have similar rarefaction curves, indicating comparable richness (seeFig. 4). Figure 3: Rarefied within sample richness based on selected fossil and extant pollen data. Curves indicate the number of expected taxa for a certain sample size (that is, number of pollen grains counted). ( a ) Curves contrasting the late Miocene (light-green curves) with present (light-blue curves) and early Miocene (orange curves) pollen assemblages from Patagonia. ( b ) Curves contrasting Patagonian (light-green curves) and Amazonian (magenta curves) pollen assemblages from the late Miocene. ( c ) Curves contrasting the Patagonian late Miocene (light-green curves) with SE Brazilian present (dark-green curves) pollen assemblages. For readability purposes, only the most diverse samples are shown. Note that the Patagonian late Miocene and SE Brazilian recent samples appear to have similar rarefaction curves, indicating comparable richness (see Fig. 4 ). 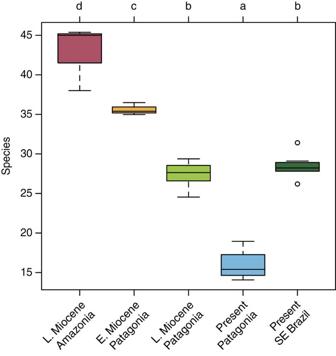Figure 4: Rarefied richness expressed as boxplots based on selected fossil and extant pollen data. The boxes delimit the first (25%) and third (75%) quartiles while the bars delimit the second (median) quartile.Post hocTukey test results are shown with different letters above each data set. Letters denote groupings based on lack of statistical difference among sequences (that is, for plot ‘L Miocene Patagonia’ and ‘Present SE Brazil’ marked ‘b’ are statistically indistinguishable from each other). Open circles represent a subset of observations (outliers) that appear to be inconsistent with the remaining data. Full size image Figure 4: Rarefied richness expressed as boxplots based on selected fossil and extant pollen data. The boxes delimit the first (25%) and third (75%) quartiles while the bars delimit the second (median) quartile. Post hoc Tukey test results are shown with different letters above each data set. Letters denote groupings based on lack of statistical difference among sequences (that is, for plot ‘L Miocene Patagonia’ and ‘Present SE Brazil’ marked ‘b’ are statistically indistinguishable from each other). Open circles represent a subset of observations (outliers) that appear to be inconsistent with the remaining data. Full size image Climatic profiles for the interval 10–6 Myr ( Fig. 5 ) indicate the extreme (minimum) temperatures and precipitation values at which our selected taxa could maintain viable populations are 11.4 °C<MTCQ>16.9 °C and 661 mm<AP>1,156 mm. 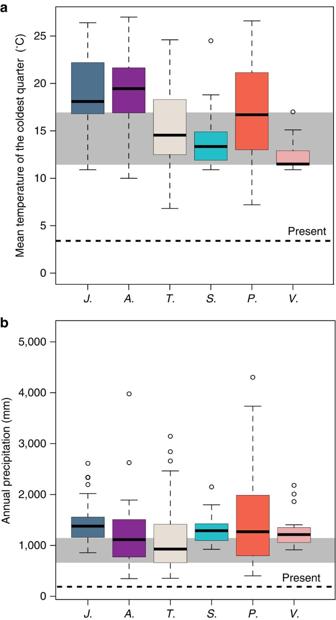Figure 5: Profiles of climatically key-sensitive species recovered in the late Miocene from Patagonia. Letters denote initials of selected genera:Justicia (J.),Achatocarpus (A.),Tripodanthus (T.), Schlechtendalia (S.),Passiflora (P.)andViviania(V.) (observeFig. 2cfor their present geographic distribution). (a) Mean Temperature of the Coldest Quarter (MTCQ) estimates for each species (Mean 15.6 °C for all species) and (b) Annual Precipitation (AP) estimates for each species (Mean 1,198 mm for all species). Horizontal dashed line represents the MTCQ and AP today in Patagonia (3.5 °C and 200 mm, respectively). Shaded grey area represents the range between the lowermost and the uppermost 25% percentile of all selected species profiles (11.4 °C<MTCQ <16.9 °C and 661 mm<AP<1,156 mm). Open circles represent a subset of observations (outliers) that appear to be inconsistent with the remaining data. Area under surves (AUCs) prediction values of the bioclimatic model range between 0.72 (Schlechtendalia, Asteraceae) to 0.81 (Tripodanthus, Loranthaceae). Values of AUC range from ≤0.5 for models with no predictive ability, to 1.0 for models giving perfect predictions49. Figure 5: Profiles of climatically key-sensitive species recovered in the late Miocene from Patagonia. Letters denote initials of selected genera: Justicia (J.) , Achatocarpus (A.) , Tripodanthus (T.), Schlechtendalia (S.) , Passiflora (P.) and Viviania ( V .) (observe Fig. 2c for their present geographic distribution). ( a ) Mean Temperature of the Coldest Quarter (MTCQ) estimates for each species (Mean 15.6 °C for all species) and ( b ) Annual Precipitation (AP) estimates for each species (Mean 1,198 mm for all species). Horizontal dashed line represents the MTCQ and AP today in Patagonia (3.5 °C and 200 mm, respectively). Shaded grey area represents the range between the lowermost and the uppermost 25% percentile of all selected species profiles (11.4 °C<MTCQ <16.9 °C and 661 mm<AP<1,156 mm). Open circles represent a subset of observations (outliers) that appear to be inconsistent with the remaining data. Area under surves (AUCs) prediction values of the bioclimatic model range between 0.72 ( Schlechtendalia , Asteraceae) to 0.81 ( Tripodanthus , Loranthaceae). Values of AUC range from ≤0.5 for models with no predictive ability, to 1.0 for models giving perfect predictions [49] . Full size image Our analysis demonstrated that the southern Andean uplift was apparently not the sole determinant force of Patagonian desertification as previously insinuated using isotopic, sedimentological or tectonic evidence [5] , [6] , [7] . Our results show that well after the assumed rain-shadow became effective (or enhanced), eastern Patagonia was covered by a significantly more diverse flora than today, comparable with that prevailing at lower (subtropical) latitudes. If the onset of Patagonian desertification was not the first-order response to the rain-shadow cast over the eastern Patagonian side, then we must seek another (and modern) explanation for this major shift. We did recognize a drop in rarefied diversity values from the early to the late Miocene (from about 50 species to 28 species). We associate this drop in richness with the extinction of several rainforest (hyper-humid) taxa, in particular several fern (for example, tree-ferns of the Cyatheaceae) and gymnosperm (for example, Dacrycarpus , Dacrydium , Lagarostrobus , Mychrocacrys ) taxa that no longer grew in eastern Patagonia since the Mid Miocene times [11] , [12] . The magnitude of this drop in diversity, however, was likely exacerbated by the fact that during late Early Miocene and Mid Miocene times an exceptionally high number of plant species was recorded in Patagonia, probably in response to a period of global warming (formally known as mid-Miocene Climatic Optimum) that culminated with the highest temperatures of the Neogene [11] , [12] , [13] . This worldwide warming event (17–14.5 Myr) appears to have favoured the expansion of tropical plant lineages into the highest latitudes of world [14] , [15] . Our late Miocene reconstructed scenario from present-day bioclimatic estimates resulted in an accurate picture of the lowest possible conditions that a selected group of taxa could have survived and reproduced (MTCQ between 11.4 °C and 16.9 °C; AP between 661 mm and 1,156 mm). Interestingly, these group of taxa (that is, Achatocarpus , Passiflora , Justicia , Tripodanthus , Viviania and Schlechtendalia ) coexist today in northeastern Argentina ( Fig. 2c ) along the Uruguay River under mesothermal (MTCQ between 14 °C and 16 °C), relatively humid (AP=1,200 mm) and windless conditions. Further palaeontological data provides additional evidence to the late Miocene estimated climate: the occurrence of fossil capybara ( Hydrochoerus hydrochaeris ) remains preserved in the studied fossil pollen-bearing deposits [16] . Today capybara extends from Venezuela to central-eastern Argentina and occupies riparian forest and seasonally flooded savannas. Also preserved in the collected sediments are fossil marine invertebrates with strong Caribbean affinities that led Martinez and del Río [17] to suggest sea surface temperatures between 20 °C and 24 °C. Our reconstructed scenario lead us to reject earlier assumptions about a late Miocene Patagonian landscape covered by needleleaf forests or grass-dominated landscapes according to climatic simulations [18] and indirect estimates [5] , respectively. Terrestrial sediments from eastern Patagonia provide another independent proxy-record to the Neogene climate, although these are mostly confined to the Early and Mid Miocene. In general, Miocene terrestrial (and terrestrial-marine transitional) exposed sediments from eastern Patagonia mainly comprise deltaic, fluvial and estuarine palaeoenvironments [19] , [20] indicating, at least, higher rainfall and freshwater runoff than today. Contrasting types of paleosols associated to fluvial deposits were recorded in Early and Mid Miocene sequences of central Patagonia, indicating some periods of aridity in a context of a general humid trend [21] . The broad ‘Patagonian’ sea [22] , [23] during the Early Miocene may have also contributed to the regional moisture in the Patagonian interior. As this inland sea contracted during the Late Miocene, it would have left the Patagonian interior more arid and would also have intensified the continentality, with warmer summers and colder winters. The expansion of open-habitat plant lineages by the late Miocene is also consistent with this change in land-sea distribution [24] . Pliocene terrestrial deposits (Río Negro Fm.) record aeolian deposits [25] suggesting probably a dryer scenario. Recent thermochronological evidence from the Patagonian Andes between 38 °S to 49 °S—latitudinal range included in our fossil collecting sites—record a marked acceleration in erosion 7–5 Myr ago (latest Miocene–Pliocene) probably triggered by the onset of a widespread Neogene glaciation in southern South America [26] . Towards higher latitudes (49 °S–56 °S), in contrast, glacial conditions prevented the erosion of the southern Andean range, leading Thomson and others [26] to recognize it as the first example of regional glacial protection of an active orogen from erosion. This glacial protection allowed the southernmost Andes to increase in height and width, probably intensifying the rain-shadow effect in the highest latitudes of the Patagonian plains by the latest Miocene–early Pliocene. It seems clear that a number of plant taxa that occupied southern South America during late Miocene times have largely been eliminated from the non-Andean regions during the last 6 million years (Pliocene-Quaternary). Others, in contrast, were uncommon during Miocene times but became dominant sometime during the Pliocene-Quaternary for the first time on these southern landscapes such as the grass family. Interestingly, a sudden increase of grassland-dominated ecosystems occurred in several regions of the earth’s land surface during Miocene times [27] . However, our results provide no evidence for major changes in grass abundance during this time interval in Patagonia ( Supplementary Table 1 ), despite the fact that the prevailing climate could have favored (C 4 -) grassland expansion. Hence, we support the view that the Miocene spread of grasslands was triggered by an episode of increased aridity affecting some regions (for example, Asia and North America) in a context of low pCO 2 conditions rather than a global-scale turnover [27] . The associated climatic conditions driven by the rain-shadow appears not to have been enough to remove other tree taxa from the present-day desert, for example Saxegothaea , Araucaria and Maytenus . Recent isopoll (equal pollen lines) maps of these three genera show that the distribution of their producers can be sharply delineated by the pollen spectrum [10] , probably because these trees produce pollen grains with limited pollen dispersal. Hence, we interpret the occurrence of these taxa as the most important elements of partially open woodland at some distance from the coast. Also, the frequent occurrence of widely dispersed pollen grains of Podocarpus and Nothofagus indicate the presence of regionally distributed forest in the late Miocene Patagonian interior. Taken all together, we strongly support the notion that the southern Andean uplift did cause a change in Patagonian landscapes, particularly because of the extinction of several rainforest lineages, dominant during early and mid Miocene times [11] , [14] , [15] . However, the climatic consequences of this uplift were not strong enough to wipe out many of the tropical and humid-demanding taxa, and even less to promote the expansion of the present grass-dominated steppe. The onset of Patagonian desertification most likely occurred during the last 6 Myr, following the Pliocene expansion of ice sheets in Antarctica [28] , the widespread Neogene glaciation of the southern Andean range [29] and the abrupt increase in wind strength (that is, westerlies) in southern mid-latitudes [30] . The initial desertification of Patagonia seems not to have been an isolated event triggered by a regional forcing but rather, part of a much widespread phase of aridity that would have also brought a full desert climate to other regions (for example, central Australia [31] and northern Chile [32] ) during the Pliocene-Pleistocene interval. Fossiliferous localities Samples were collected from the Puerto Madryn (42°34′39′′S; 64°16′35′′W) and Barranca Final (40°54′38′′S; 64°25′14′′W) formations. The former consists of 150 m of sandstone, heterolithic and bioclastic beds [33] that crop out mainly along the coasts of the Valdes Peninsula, in northeastern Patagonia ( Fig. 2c ). These sediments were deposited in open marine to tide-dominated estuarine environments [34] . Samples consist of fine-grained deposits taken near the base of the section ( Fig. 6 ) in what del Río et al. [35] called the Maximum High-stand Phase, which is the deepest part of the sedimentary system. The age of the Puerto Madryn Formation (Fm.) was calibrated by 87 Sr/ 86 Sr ratios on calcitic shells at about 10 Myr (Tortonian) [33] . Outcrops of the Barranca Final Fm. are limited to a narrow and thin (about 15 m) belt of cliffs in the northern coast of the San Matías Gulf, where its type locality is located [34] . There, it is composed of fossiliferous dark claystone, siltstone and fine sandstone beds, deposited in a protected, low-energy shallow marine/estuarine environment. The lower contact is not visible and the upper contact is gradational to the overlying terrestrial Río Negro Fm. ( Fig. 6 ). We sampled three entire well-preserved oyster valves for 87 Sr/ 86 Sr isotopic analysis of the shell carbonate. Each valve was cut and polished ( Supplementary Fig. 2 ) for microsampling following the criteria established by Cuitiño et al. [36] . From each valve ~30 mg of carbonate powder was obtained with a dental drill. Chalky microstructures were avoided because these are susceptible to diagenetic alteration [36] . 87 Sr/ 86 Sr isotopic analyses were performed with a Neptune ICP Mass Spectrometer at the Geochronos Laboratory of the University of Brasilia, Brazil. Age calculations are based on the Look-Up Table of McArthur et al. [37] with an uncertainty of 0.07 Myr derived from the mean curve. The three obtained ages correspond to the late Miocene interval (9.61, 8.3 and 6.48 Myr). Dinoflagellate cyst stratigraphy provides additional age control for the Miocene from northeastern Patagonia ( Supplementary Note 1 ). 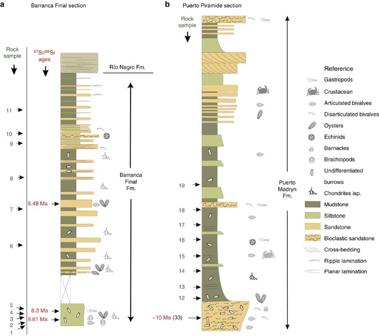Figure 6: Stratigraphic logs of the studied sections. Sedimentary features,87Sr/86Sr ages and rock sampling levels are shown for the two studied localities (vertical scale: 1:200). The Barranca Final section shows an upward continentalization, evidenced by the reduction in the abundance of marine fossils and ichno- fossils as well as marine dinocyst species. The lowermost layers contain the most diverse marine macro and microfossil association suggesting connection to the open ocean whereas the mid levels represent low-energy estuarine to coastal lagoon environments, that experienced reduced oxygenation episodes evidenced by monospecific layers of the ichnofossilChondritesisp. The sedimentary system grades upward to terrestrial sandstones and mudstones of the Río Negro Formation (Fm.). For the southern Puerto Madryn Fm. only the basal, palynologically-productive part of the Puerto Pirámide section is represented. The stratigraphic phases correspond to del Ríoet al.35. According to del Ríoet al.35the Maximum High-stand Phase is the deepest (inner-mid shelf) phase achieved by the sea during the deposition of this unit.87Sr/86Sr ages for different parts of this unit are around 10 Myr33. Figure 6: Stratigraphic logs of the studied sections. Sedimentary features, 87 Sr/ 86 Sr ages and rock sampling levels are shown for the two studied localities (vertical scale: 1:200). The Barranca Final section shows an upward continentalization, evidenced by the reduction in the abundance of marine fossils and ichno- fossils as well as marine dinocyst species. The lowermost layers contain the most diverse marine macro and microfossil association suggesting connection to the open ocean whereas the mid levels represent low-energy estuarine to coastal lagoon environments, that experienced reduced oxygenation episodes evidenced by monospecific layers of the ichnofossil Chondrites isp. The sedimentary system grades upward to terrestrial sandstones and mudstones of the Río Negro Formation (Fm.). For the southern Puerto Madryn Fm. only the basal, palynologically-productive part of the Puerto Pirámide section is represented. The stratigraphic phases correspond to del Río et al. [35] . According to del Río et al. [35] the Maximum High-stand Phase is the deepest (inner-mid shelf) phase achieved by the sea during the deposition of this unit. 87 Sr/ 86 Sr ages for different parts of this unit are around 10 Myr [33] . Full size image Pollen sampling and processing We collected 143 pollen samples from the Puerto Madryn and Barranca Final formations during several summer field-trips. Our palynological record is well constrained and is not hampered by facies changes typical for the terrestrial environment. Forty-eight samples yielded palynomorphs from which we selected beds containing landscape-level pollen representation (mostly estuarine and shallow marine facies), in which usually marine dinoflagelate cysts as well as river-and wind-transported terrestrial specimens occur. The material recovered is very well preserved, making taxonomic assignments valuable and accurate. Standard processing techniques of recovering palynomorphs were employed [38] . Two hundred pollen and spores—when possible—were counted per sample. An important number of counted specimens correspond to wind-pollinated (anemophilous) taxa (that is, largely southern beech and podocarp pollen grains in southern South America). This can mislead the interpretation about what type of flora (and associated climate) occurred near the accumulation site because pollen grains produced by most anemophilous taxa are widely dispersed. We hence based our climatic inferences on those fossil pollen types likely to have been dispersed short distances from the parent plants (that is, mainly entomophilous taxa). Quantitative analysis We conducted all analyses using the open-source software R (The R Project for Statistical Computing, version 3.0.1). We arranged pollen data in a matrix with samples and taxa in which each cell contained count data for all taxa of the selected samples ( Supplementary Table 1 ). We estimated within-sample diversity using rarefaction because the count sizes for the samples slightly differed. Differential count sizes will bias any estimate of within-sample diversity as larger count sizes correspond to greater richness within a sample [39] . Rarefaction allowed us to down-sample those larger samples until they are the same size as the smallest sample [40] , making fair comparisons between incomplete samples. We estimated rarefaction using rarefy function of the R’s community ecology package ‘vegan’ [41] and compared sample diversity at 185 grains because all samples have at least this number of counted pollen–spore specimens. We compared rarefied richness to fossil and/or recent assemblages from elsewhere in South America. Among all pollen matrixes obtained for comparison (either fossil or recent), we only selected those with the best taxonomic resolution possible. For example, we did not consider matrixes containing the variable Asteraceae as the sole taxonomic member of this eurypalinous family. Raw count data matrixes were either received via e-mail by the authors of their respective palynological contributions or obtained from our published palynological results. We selected pollen–spore raw count data for the: (a) mid-late Miocene Pebas Fm. (Mocagua section, three samples) from Colombia (70°17′W; 3°48′S), Amazonian region [42] , (b) early Miocene Chenque Fm. (Baumann section, three samples) from southern Argentina, Patagonian region [43] , (c) Pleistocene (Gelasian, one sample) section from central Patagonia [24] , (d) present pollen-rain (five samples) samples from Rio Grande do Sul (28°56′16″, 50°02′39.9″W), southeastern Brazilian region [44] and (e) present pollen-rain (four samples) from northeastern Patagonia, very close to the fossil collecting site [45] . Differences in rarefied species richness were tested among all of these South American spore–pollen assemblages using analysis of variance (ANOVA). We tested normality (Shapiro–Wilk test) before running ANOVA. We then used a Tukey test to identify which groups were statistically different from each other. Paleoclimate estimation The reliability and resolution of the ‘Coexistence approach’—widely used to reconstruct past climates using fossil plant data—has been examined in detail by Grimm & Denk [46] . These authors severely criticized this method and encouraged palaeontologists to use the minimum tolerances of the nearest living relatives instead. We hence estimated the minimum temperature and precipitation values at which a selected number of climate (drought and frost)-sensitive species are suitable to maintain viable populations. These selected taxa—recognized from the fossil pollen types described and illustrated here ( Supplementary Note 2 ; Supplementary Fig. 3 )—include Schlechtendalia luzulaefolia (Asteraceae), Justicia laevilinguis (Acanthaceae), Viviania albiflora (Vivianiaceae), Achatocarpus spp. (Achatocarpaceae), Tripodanthus acutifolius (Loranthaceae) and Passiflora spp. (Passifloraceae). These taxa have never been recorded in older Miocene deposits [11] nor in recent botanical expedition in Patagonia; therefore, we reject the possibility of pollen recycling from older deposits or contamination from recent parent plants. With the aim of estimating the lowest minimum temperature and precipitation values, we first downloaded geo-referenced data of those selected species from the Global Biodiversity Inventory Facility portal ( www.gbif.org ). We removed duplicated points using the R’s package ‘base’ (function ‘duplicated’) and then plotted the occurrence data using the R’s package ‘maptools’ (function ‘wrld_simpl’) to eliminate misplaced points (for example, points in the ocean). We then extracted bioclimatic variables—that is, parameters that are biologically meaningful combinations of monthly climate data [47] —of the point locations from the WorldClim database ( http://www.worldclim.org , 10’ resolution) using the Bioclimatic envelope model as implemented in the R’s package Dismo [48] . This model uses associations between aspects of climate and species’ occurrences to estimate the conditions that are suitable to maintain viable populations [49] . The two selected limiting variables were MTCQ and AP. We defined the range of the lower climatic limits using the 25 percentile of all species envelopes to provide a tight climatic profile. We conducted a model evaluation by means of area under curve statistics from a receiver-operating characteristic analysis [48] , which is—in the context of Dismo package–a rank-correlation test. How to cite this article: Palazzesi, L. et al. Fossil pollen records indicate that Patagonian desertification was not solely a consequence of Andean uplift. Nat. Commun. 5:3558 doi: 10.1038/ncomms4558 (2014).